Scaling laws for van der Waals interactions in nanostructured materials Van der Waals interactions have a fundamental role in biology, physics and chemistry, in particular in the self-assembly and the ensuing function of nanostructured materials. Here we utilize an efficient microscopic method to demonstrate that van der Waals interactions in nanomaterials act at distances greater than typically assumed, and can be characterized by different scaling laws depending on the dimensionality and size of the system. Specifically, we study the behaviour of van der Waals interactions in single-layer and multilayer graphene, fullerenes of varying size, single-wall carbon nanotubes and graphene nanoribbons. As a function of nanostructure size, the van der Waals coefficients follow unusual trends for all of the considered systems, and deviate significantly from the conventionally employed pairwise-additive picture. We propose that the peculiar van der Waals interactions in nanostructured materials could be exploited to control their self-assembly. The discovery and the ensuing burst of applications of carbon-based nanomaterials, including fullerenes [1] , carbon nanotubes [2] , single-layer and multilayer graphene (MLG) [3] , have undoubtedly revolutionized materials science, revealing bright prospects in nanotechnology and other related fields. Low-dimensional nanostructures have been demonstrated to possess previously unexpected electronic [4] , optical [5] , cohesive [6] , [7] and thermal [8] properties. The self-assembly of such nanostructures is often governed by the ubiquitous van der Waals (vdW) interactions, the description of which requires the usage of quantum electrodynamics [9] , [10] . Despite this well-known fact, most of the widely employed atomistic models for vdW interactions in nanomaterials are based on a simple pairwise interacting ‘atoms-in-molecules’ picture, ignoring the rather strong electrodynamic response effects, which stem from long-range fluctuations in matter. Recent work by Ruzsinszky et al. [7] showed that electrodynamic effects can dramatically influence the vdW interaction between large fullerene molecules. Here we determine the microscopic polarizability and vdW coefficients of molecules and materials, including electrodynamic response effects, by utilizing a recently developed parameter-free method based on a system of coupled quantum harmonic oscillators (QHO) [11] . This method is applied to a wide range of carbon-based nanomaterials, including fullerenes, carbon nanotubes and nanoribbons, graphite, diamond, as well as single-layer and MLG. Our microscopic calculations, valid at close and far (<10 nm) separations between nanostructures, reveal that vdW interactions act at distances greater than typically assumed and show unusual behaviour depending on the dimensionality of the system. The peculiar vdW scaling laws lead to a decreasing binding energy for a fullerene molecule adsorbed on MLG as a function of the number of graphene layers, contrary to conventional expectations. Calculation of vdW coefficients Here only the salient features of our method are described. We refer the reader to ref. 11 and the Methods section for additional details of our approach. We map a given molecule or material to a system of QHO, with a single QHO assigned to every atom. The QHO parameters are determined as functionals of the ground-state electron density, obtained from density-functional theory (DFT) calculation of the self-consistent electronic structure, using the Tkatchenko–Scheffler (TS) method [12] . The QHOs are subsequently coupled through the dipole–dipole potential, and the response of the fully interacting many-atom system is determined upon solving the self-consistent Dyson-like screening equation [13] , [14] , [15] . The solution of the self-consistent screening (SCS) equation yields the interacting frequency-dependent polarizability for the system of interest, thus going beyond the standard pairwise approximation. The fundamental equations of the employed method are equivalent to ref. 11 , with an improved mapping of the interactions present in the full electronic system to the QHO model. This simple yet effective modification leads to a noticeable improvement in the description of the static polarizability for molecules and solids. vdW coefficients of model systems Before applying our method to carbon nanostructures, we investigated its performance for fundamental carbon-based model systems: benzene, C 60 fullerene, graphite and diamond. For the polarizability and vdW C 6 coefficients of small molecules, such as benzene, the conventional ‘atoms-in-molecules’ picture can be successfully employed. For example, the TS method [12] leads to accurate values of α =74.4 bohr 3 and C 6 =1,783 hartree· bohr 6 for benzene, compared with reference experimental values of α =71.3 bohr 3 and C 6 =1,723 a.u. [16] , [17] (here and in what follows, the notation ‘a.u.’ is used to denote Hartree atomic units). However, the TS method does not capture the anisotropy in the polarizability [11] , which arises mainly from the interaction between the dipoles. Upon including the electrodynamic response by solving the SCS equation, the anisotropy in the static polarizability is significantly improved, whereas the isotropic vdW C 6 coefficient is still accurately determined (1,697 a.u.). Predicting accurate polarizability and C 6 coefficient for the C 60 fullerene is a more demanding task because of the coupling between localized sp 2 bonds and excitations delocalized over the C 60 molecule. The experimental estimate for the static polarizability of C 60 is 8.6±0.9 a.u. per atom [18] . The SCS method somewhat underestimates the static polarizability and yields 7.5 a.u. per atom. This is consistent with the fact that the inclusion of excitations delocalized over the whole molecule will increase the static polarizability of the C 60 molecule. However, here our focus lies on the C 6 coefficients, which are obtained upon integration over the imaginary frequency. The ‘metal-like’ delocalized excitations become important only at rather low imaginary frequencies, and their inclusion is not expected to appreciably change our conclusions. In fact, the computed carbon–carbon C 6 coefficient of 24.2 a.u. inside C 60 is only slightly lower than the time-dependent hybrid DFT (TDDFT) estimate of 28.3 a.u. [19] , [20] . Similarly accurate results are obtained for solids, including graphite and diamond. For graphite, we determine the C 6 coefficient of 28 a.u., which is in good agreement with the estimate done using the experimentally measured dielectric function (24 a.u.) [21] . For diamond, the computed value of 22 a.u. agrees rather well with the value of 17 a.u. determined from the experimental dielectric function [22] . We conclude that our method is capable of accurately describing the frequency-dependent polarization and the resulting vdW C 6 coefficients for a wide range of molecules and solids. We proceed to study the vdW C 6 coefficients for carbon nanostructures of different dimensionality. vdW coefficients of carbon nanostructures The main results are summarized in Fig. 1 , where we present the C 6 coefficient per carbon atom (see definition in the Methods section) for nanostructures of different dimensionality, including zero-dimensional fullerenes, one-dimensional single-wall carbon nanotubes, two-dimensional single-layer and MLG, and three-dimensional graphite and diamond. The C 6 coefficient per carbon atom varies by almost an order of magnitude among the different nanostructures, with the lowest value found for small fullerenes and the largest for graphene. These findings demonstrate that the conventional approximation of fixed carbon–carbon C 6 coefficient fails dramatically when modelling vdW interactions between nanostructures. The pairwise approximation is especially problematic when the interaction between different nanostructures is studied, for example, binding between fullerenes/nanotubes with graphene layers or graphite surface (see below). 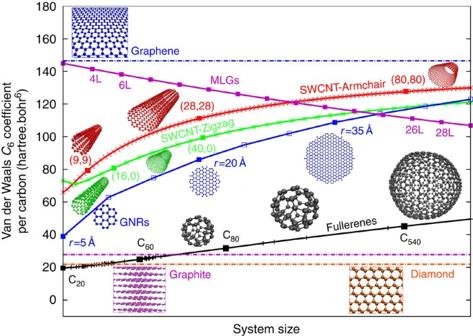Figure 1: Scaling laws for vdW coefficients. vdWC6coefficients per carbon atom (theC6of the full system divided byNC2, whereNCis the number of carbon atoms) for nanostructures of different dimensionality, as calculated by the electrodynamic response model of ref.11. The size ranges for different systems are as follows: (1) the radius of fullerenes is varied from 2 to 12 Å; (2) the radius of single-wall carbon nanotubes (SWCNT)-Armchair(n,n) and SWCNT-Zigzag(n,0) vary between 2 and 60 Å; (3) the graphene nanoribbons (GNRs) vary in radius from 5 to 50 Å; (4) the number of layers in multilayer graphene (MLG) varies from 2 to 30, where each point on the plot corresponds to an increase of two layers. Figure 1: Scaling laws for vdW coefficients. vdW C 6 coefficients per carbon atom (the C 6 of the full system divided by N C 2 , where N C is the number of carbon atoms) for nanostructures of different dimensionality, as calculated by the electrodynamic response model of ref. 11 . The size ranges for different systems are as follows: (1) the radius of fullerenes is varied from 2 to 12 Å; (2) the radius of single-wall carbon nanotubes (SWCNT)-Armchair( n , n ) and SWCNT-Zigzag( n ,0) vary between 2 and 60 Å; (3) the graphene nanoribbons (GNRs) vary in radius from 5 to 50 Å; (4) the number of layers in multilayer graphene (MLG) varies from 2 to 30, where each point on the plot corresponds to an increase of two layers. Full size image We proceed to analyse the C 6 per carbon atom as a function of system size for different classes of nanostructures. For the fullerene family, the system size is defined by the fullerene radius. Therefore, as shown in Fig. 1 , the C 6 coefficient increases linearly as a function of the fullerene radius. This leads to the following fitted scaling power law as a function of the number of carbon atoms n , ≈ n 2.35 . In contrast, a simple parwise approximation predicts ≈ n 2 . The faster growth of C 6 coefficients upon including electrodynamic response can be explained by the polarization (depolarization) inside the fullerene (vacuum) when increasing the fullerene radius. In fact, in the limit of giant fullerenes, the C 6 per carbon should approach that of a carbon atom in a graphene layer. However, local curvature effects clearly reduce the polarizability even for quite large fullerenes. The rapid increase of C 6 is in qualitative agreement with recent calculations based on a representation of a fullerene as a hollow metallic sphere, in which it was found that in the asymptotic regime of giant fullerenes, grows as n 2.75 (ref. 7 ). The smaller exponent found in our work stems from a fit to smaller fullerene sizes and from the fact that every carbon atom is modelled as a QHO. We consider this atomistic representation as more realistic compared with modeling fullerenes as hollow metallic spheres. In fact, recent TDDFT calculations suggest a scaling power law of ~ n 2.2 for of fullerenes from C 60 to C 84 (ref. 20 ). Our model yields a very good agreement with TDDFT for these small fullerenes, predicting a scaling of ~ n 2.25 . In conclusion, three different methods unambiguously demonstrate that the coefficient grows much faster in fullerenes than a simple pairwise model would suggest. For graphene nanoribbons (GNRs), the system size is defined by the radius of the circle enclosing the GNR. In contrast to fullerenes, the C 6 coefficients of GNRs increase superlinearly as a function of the GNR radius. There are significant edge-polarization effects in GNRs, which lead to larger polarizability density as one goes away from the centre of the GNR towards the edges. This behaviour is explained by stronger polarization of ‘less constrained’ edge atoms. As expected, the C 6 coefficients of GNRs tend to that of single-layer graphene as the GNR size grows. Similar to the case of GNRs, the C 6 coefficients of single-walled carbon nanotubes (SWCNTs) grow superlinearly as a function of the SWCNT radius. The vdW coefficients also depend on the chirality of the SWCNTs, in general increasing faster for armchair nanotubes than for zigzag ones. The superlinear increase of the C 6 coefficient for SWCNTs stems from the remarkable axial polarization that arises from the favourable alignment of the dipoles along the SWCNT axis. In contrast, we find depolarization in the direction perpendicular to the SWCNT. Both of these findings are in agreement with DFT calculations [23] . However, our method is significantly more efficient and allows the calculation of the microsopic polarization tensor even for very large nanostructure assemblies containing many thousands of atoms. Not unexpectedly, even more remarkable behaviour is noticeable for single-layer graphene and MLG nanostructures. The carbon–carbon C 6 coefficient of 147 a.u. in two-dimensional graphene is 5.3 times larger than that of three-dimensional graphite. This can be rationalized by a substantial in-plane polarization in graphene on the expense of depolarization in the direction perpendicular to the graphene layer. In contrast, the interplay of interlayer and intralayer polarization leads to a smaller C 6 coefficient for carbon in graphite. Notably, the convergence of the C 6 coefficient from the graphene limit to the graphite limit is exceedingly slow as a function of the number of graphene layers for MLGs. We observe a linear behaviour for up to 30 stacked graphene layers, and a naive linear extrapolation suggests that at least 90 graphene layers would be required to converge the carbon–carbon C 6 coefficient to the graphite limit. From the geometry point of view, such an unusually slow convergence stems from noticeable surface polarization effects for MLGs. Physically, this behaviour can be explained by the self-consistent nature of electrodynamic response equations that effectively couple all the interacting QHOs, leading to effects that propagate much further beyond the decay of the standard dipole–dipole ~ interaction law, where R AB is the distance between two QHOs. vdW binding between carbon nanostructures Having presented the peculiar scaling laws for vdW coefficients in different carbon nanostructures, we now study the impact of our findings for the interlayer-binding energy in graphite and the C 60 fullerene interacting with MLGs. The interlayer-binding energy of graphite has been a subject of intense investigation over the last decade. Experimental measurements yield values from 31±2 meV (ref. 24 ) to 52±5 meV (ref. 25 ) per carbon atom. State-of-the-art theoretical calculations using the random-phase approximation (utilizing Perdew–Burke–Ernzerhof (PBE) [26] wavefunctions) to the electron correlation energy predicts a value of 48 meV per atom [27] , whereas quantum Monte Carlo calculations yield a larger value of 56 meV per atom [28] . The interlayer binding in graphite has been frequently approximated as a sum of pairwise potentials with vdW C 6 coefficients obtained using the experimental dielectric function of graphite (24 a.u.) or explicitly fitted to experimental measurements. Such a simple approximation assumes that the carbon–carbon C 6 coefficient is the same in graphene and graphite, and this result is far from reality as clearly illustrated in Fig. 1 . Electrodynamic response effects lead to radically different polarization behaviour in two-dimensional graphene and three-dimensional graphite. In Fig. 2 , the interlayer-binding energy of graphite is presented as a function of the distance between the layers. The pairwise approximation using the PBE-TS method [12] overestimates the binding considerably, by at least 30 meV per atom. Accurate inclusion of electrodynamic response screening in the PBE-TS+SCS [22] method leads to interlayer-binding energy that agrees exceptionally well with the measurements of Zacharia et al. [25] , as well as random-phase approximation [27] and quantum Monte Carlo [28] calculations. The important improvement of the binding energy in the PBE-TS+SCS method stems from a much larger C 6 coefficient of graphene when compared with graphite. This results in an increased vdW energy contribution for a carbon atom inside graphene and a concomitantly smaller interlayer-binding energy. 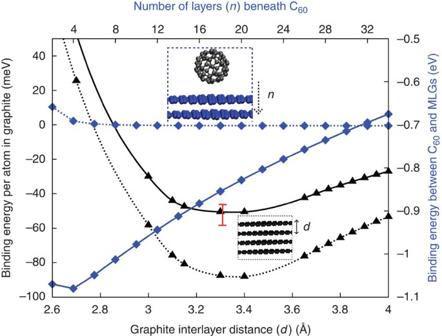Figure 2: vdW binding between nanostructures. Graphite interlayer-binding energy as a function of the interlayer distancedusing the PBE functional with TS pairwise vdW energy (PBE-TS, dotted black line, triangles) and PBE with self-consistently screened (SCS) vdW energy (PBE-TS+SCS, solid black line, triangles). The measured experimental-binding energy from ref.25is marked in red. Binding energy of C60fullerene on multilayered graphene as a function of number of graphene layers, using PBE-TS (dotted blue line, diamonds) and PBE-TS+SCS (solid blue line, diamonds) methods. The centre of the C60molecule is located 7.5 Å away from the closest graphene sheet. Figure 2: vdW binding between nanostructures. Graphite interlayer-binding energy as a function of the interlayer distance d using the PBE functional with TS pairwise vdW energy (PBE-TS, dotted black line, triangles) and PBE with self-consistently screened (SCS) vdW energy (PBE-TS+SCS, solid black line, triangles). The measured experimental-binding energy from ref. 25 is marked in red. Binding energy of C 60 fullerene on multilayered graphene as a function of number of graphene layers, using PBE-TS (dotted blue line, diamonds) and PBE-TS+SCS (solid blue line, diamonds) methods. The centre of the C 60 molecule is located 7.5 Å away from the closest graphene sheet. Full size image Finally, we illustrate how the peculiar scaling laws for vdW coefficients in nanomaterials can lead to unusual binding behaviour between nanostructures of different dimensionality. The binding energy of a fullerene on MLGs is shown in Fig. 2 as a function of number ( n ) of graphene layers beneath the fullerene. Conventionally, one would expect the binding energy to increase with n , as shown by the dotted blue curve in Fig. 2 , as there are more atoms to interact with (presumably equal to more polarization). In addition, a simple pairwise model would lead to a quick convergence of the binding energy with respect to n because of a rather quick decay of the pairwise vdW energy for two atoms A and B. This simple view is, however, deceptive. In fact, as n increases, the polarizability and C 6 per carbon atom in MLGs decrease (see Fig. 1 ). This leads to overall depolarization of the fullerene/MLG complex, and shows a decreasing binding energy with increasing n . As the convergence of the C 6 coefficient with n is rather slow, the binding energy also converges slowly. We remark that a fully anisotropic treatment of the vdW interactions is probable to decrease the slope of the binding energy curve for C 60 on MLGs. However, it is noteworthy that the pairwise and the fully screened vdW energy converge to different values of the binding energy, with the latter yielding somewhat weaker binding. This is consistent with our observations for the graphite interlayer-binding energy. We are not aware of direct experimental measurements for the binding energy of fullerene with graphite; however, we expect similar findings as for the graphite interlayer binding, where the PBE-TS+SCS method yields more accurate results than a simple pairwise approximation to the vdW energy. The rather unconventional behaviour of the binding energy for adsorption on MLGs with the number of layers n is a general phenomenon for a variety of adsorbates, ranging from small molecules to larger objects. To place our findings in the broader context of current understanding of vdW interactions, we note that it is widely accepted that these interactions are inherently non-additive (many-body) phenomena, corresponding to correlations between fluctuating multipoles in matter [9] . Interested readers are referred to the previous papers by Axilrod and Teller [29] , Bade [30] and Zwanzig [31] for the analysis and explanations of many-body contributions to vdW interactions. The seminal ideas proposed in this previous work to treat vdW interactions beyond simple pairwise additivity have been utilized more recently to study model systems, characterized by point polarizabilities, see for example, the analysis by Cole [32] , Donchev [33] and Dobson [34] among others. The crucial idea of our method is to extend the description from point-polarizable fluctuating dipoles to QHO extended in space and described by dipole density distributions (see Methods and ref. 35 ). All the necessary parameters are determined from the self-consistent electron density using state-of-the-art electronic structure calculations, apart from the available high-level reference data for atomic polarizabilities [11] . The efficiency and accuracy of our methods make it possible to carry out calculations on a broad variety of real materials. Recently, our methods have been implemented in the widely used VASP code [36] and benchmarked for a set of pristine three-dimensional solids. In this work, we significantly extend previous observations on the importance of electrodynamic response effects to more general nanostructures of lower dimensionality, including the interaction between different nanostructures. The coupled QHO model assumes that the material can be initially partitioned into well-defined atomic fragments. Thus, the possibility of hopping of electrons over long distances is neglected. The coupling of screening and such delocalized electrons can lead to other types of non-additivity not addressed in this work. For example, Dobson et al. [6] and Misquitta et al. [37] have identified peculiar asymptotic power laws for the interaction between low-dimensional materials. Subsequently, it has been found that these effects contribute very little at equilibrium separations between nanostructures [27] . The incorporation of delocalized electrons into the coupled QHO model will be a subject of future work. In conclusion, we have identified an unusual behaviour caused by electrodynamic response in vdW interactions for nanostructured materials. Depending on the dimensionality and the atomic arrangement of carbon atoms, the vdW coefficients per carbon atom exhibit peculiar scaling laws that can be exploited for controlling the self-assembly of complex nanostructures, as recently suggested by experimental measurements [38] , [39] . Calculation of the non-local polarizability tensor The long-range non-retarded vdW energy between two atoms in vacuo originates from the electrodynamic interaction of ‘atomic’ dipolar fluctuations. However, when an atom is embedded in a condensed phase (or in a molecule), the corresponding dipolar fluctuations significantly differ from the free-atom case, and in fact, this difference originates from both the local chemical environment surrounding the atom and the long-range electrodynamic interaction with the more distant fluctuating dipoles decaying via a ~1/ R 3 interaction law. Depending on the underlying topology of the chemical environment, this fluxional internal electric field can give rise to either polarization or depolarization effects, and is largely responsible for the anisotropy in the molecular polarizability tensor [14] , [15] . To address these non-additive effects, we represent the N atoms in a given material as a collection of N QHO, each of which is characterized initially by an isotropic frequency-dependent dipole polarizability. To account for the local chemical environment, we utilize the TS prescription [12] , in which the static polarizability [ n ( r )] and the excitation frequency [ n ( r )] for every i -th QHO are defined as functionals of the ground-state electron density n ( r ) obtained from a self-consistent quantum mechanical calculation using DFT. We require that the response of the material is not dominated by delocalized excitations and can therefore be initially divided into effective atomic fragments. The Hirshfeld [40] partitioning of the electron density is then utilized to account for the local chemical environment surrounding each atom. As both parameters ( [ n ( r )] and [ n ( r )]) are referenced to highly accurate free-atom reference data, short-range quantum mechanical exchange-correlation effects are accounted for in these quantities by construction. In fact, the frequency-dependent polarizabilties defined in this manner yield C 6 coefficients that are accurate to 5.5% when compared with reference experimental values for an extensive database of atomic and (small) molecular dimers [12] . To accurately capture the long-range electrodynamic response screening and anisotropy effects beyond the local chemical environment, we self-consistently solve the Dyson-like screening equation (SCS), see equations (2)–(4), in ref. 11 . In short, we solve the following equation to determine the non-local (interacting) polarizability tensor ( r , r′ ; iω ); p and q label the Cartesian tensor components) where is the dipole–dipole interaction tensor (Hartree atomic units have been used throughout). The above SCS equation can be written as a system of algebraic equations on the basis of QHO positions, see equations (2)–(4), in ref. 11 . The interacting polarizability tensor is obtained upon solving this system of algebraic equations, and in practice amounts to an inversion of a 3 N × 3 N matrix at every frequency of interest. The charge density distribution of each QHO required for the calculation of is defined as in which σ represents the width of the Gaussian [35] . An improvement of the TS+SCS method published in ref. 11 is used for all the results reported in this paper. The parameter corresponding to every free atom i is obtained from the electron density computed with the coupled-cluster singles and doubles method by fitting the dipole potential resulting from this accurate electron density to a model QHO potential. This allows us to reliably model interactions for interatomic distances beyond ~0.5 Å. For an atom in a material, and for each frequency of the electric field, the σ parameter is defined by the aforementioned TS prescription as where is the Hirshfeld volume ratio between an atom-in-a-material and the free atom. This straightforward modification of the TS+SCS method leads to an improved performance for molecular static polarizabilities (7% mean absolute error on >7,000 organic molecules from a database used in ref. 41 ). The reference polarizabilities were calculated by applying a finite electric field to DFT calculations using the hybrid PBE0 functional. This approach yields an accuracy of 3% for polarizabilities in comparison with experimental data and high-level linear-response coupled-cluster calculations including single and double excitations. The values of the employed parameters were obtained from coupled-cluster singles and doubles calculation for the free carbon atom and DFT electron density calculations for all materials, and they are =1.514 bohr, =0.911 for the carbon atom in diamond, =0.884 for graphite and =0.863 for sp 2 -bonded carbon in all the other materials (slight variations of this value are observed in different nanostructures but these variations have negligible effect on the final results). Computation of atom–atom C 6 coefficients The total isotropic frequency-dependent polarizability for a system S is obtained upon contraction of the non-local polarizability tensor . The usual Casimir–Polder integral over polarizability at imaginary frequency is then utilized to compute the coefficient for a system S . As we are only concerned with carbon atoms in this work, the coefficient (‘per carbon atom’) is defined as / , where N C is the total number of carbon atoms in the system (or per unit cell). DFT calculations All DFT calculations have been performed using the full-potential all-electron code FHI-aims [42] . FHI-aims uses a real-space grid representation for the Kohn–Sham wavefunctions; therefore, both periodic and non-periodic systems can be treated efficiently and on equal footing (see http://www.aimsclub.fhi-berlin.mpg.de for a detailed description of the FHI-aims code). We employed the PBE functional [26] for all DFT calculations. Special care has been taken to use sufficiently large supercells to eliminate any possible interactions with artificial periodic images for low-dimensional systems. Typically, vacuum sizes of 500 Å were used for this purpose. Such large unit cells do not substantially increase the computational cost in real-space DFT codes because there are no basis functions in the vacuum region. For molecular systems (fullerenes, GNRs), no periodic boundary conditions were used. The geometries employed in this work were constructed using the experimental carbon–carbon distances for the different systems. How to cite this article: Gobre, V. V. and Tkatchenko, A. Scaling laws for van der Waals interactions in nanostructured materials. Nat. Commun. 4:2341 doi: 10.1038/ncomms3341 (2013).